Angiotensin II plasma levels are linked to disease severity and predict fatal outcomes in H7N9-infected patients A novel influenza A (H7N9) virus of avian origin emerged in eastern China in the spring of 2013. This virus causes severe disease in humans, including acute and often lethal respiratory failure. As of January 2014, 275 cases of H7N9-infected patients had been reported, highlighting the urgency of identifying biomarkers for predicting disease severity and fatal outcomes. Here, we show that plasma levels of angiotensin II, a major regulatory peptide of the renin–angiotensin system, are markedly elevated in H7N9 patients and are associated with disease progression. Moreover, the sustained high levels of angiotensin II in these patients are strongly correlated with mortality. The predictive value of angiotensin II is higher than that of C-reactive protein and some clinical parameters such as the PaO 2 /FiO 2 ratio (partial pressure of arterial oxygen to the fraction of inspired oxygen). Our findings indicate that angiotensin II is a biomarker for lethality in flu infections. The avian influenza pandemic poses a potentially grave public health threat because of the high mortality rates observed in infected people [1] , [2] , [3] , [4] , [5] . Generally, the numbers of cases from single hospitals are limited and insufficient for statistical analysis [6] . As a result, no biomarker that predict disease progression and outcomes of potentially lethal flu infections has been identified [7] . During the spring of 2013, a novel and highly virulent avian-origin influenza A subtype virus, H7N9, emerged and spread among humans in Eastern China [5] , [8] , [9] , [10] . In total, 144 people were infected by the end of 2013, and there were already over 100 newly infected patients before the end of January in 2014. Of the 111 patients we previously studied in 2013, 76.6% were admitted to an intensive care unit [1] . Among these patients, more than 70% developed acute respiratory distress syndrome (ARDS) [1] , which was associated with high mortality, as few interventions were available [11] , [12] . Although extensive therapeutic interventions were employed, including antiviral treatments, oxygen therapy, mechanical ventilation, antibiotics, glucocorticoids, intravenous immunoglobulins, extracorporeal membrane oxygenation, continuous renal replacement therapy and artificial liver support system therapy, we observed high mortality rates among H7N9-infected patients [1] , [13] , [14] , [15] . Our previous studies on sepsis, aspiration and severe acute respiratory syndrome coronavirus-induced ARDS demonstrated that dysfunction of the renin–angiotensin system (RAS) is involved in the molecular pathogenesis of ARDS [16] , [17] . In essence, angiotensin-converting enzyme (ACE) 2 and angiotensin II type 2 receptor protect mice from ARDS, whereas ACE, angiotensin II, and angiotensin II type 1a receptor promote the impairment of lung function in mouse models [16] , [17] . Moreover, in our accompanying paper [18] , we show that ACE2-mutant mice die more rapidly after H5N1 infection and that recombinant ACE2 can partially protect mice from lethal H5N1 infection. For the first time, we have gained access to samples from a large cohort of H7N9-infected patients. Therefore, we asked whether dysfunction of the RAS is present in H7N9-infected patients. Here, we report that there is a highly positive linear association between plasma levels of angiotensin II in H7N9-infected patients and disease severity scores (Acute Physiology and Chronic Health Evaluation II, APACHE II) [19] , [20] , and that angiotensin II levels can predict fatal outcomes. Elevated angiotensin II levels may reflect disease outcomes We collected plasma from 47 H7N9-infected patients who were diagnosed in Hangzhou (40), Nanjing (6) and Shanghai Autonomous City (1), China ( Supplementary Fig. 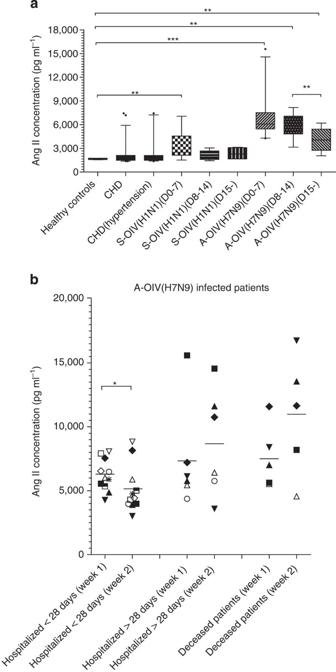Figure 1: Angiotensin II levels are increased in plasmas of H7N9-infected patients. Among the study participants, 46 patients were infected with avian-origin H7N9 Influenza A virus (A-OIV H7N9) and 21 were infected with swine-origin H1N1 influenza A virus (S-OIV H1N1). In addition, six healthy volunteers, 46 CHD patients and 35 CHD patients with hypertension were recruited as controls. (a) Angiotensin II levels in plasma of healthy controls, CHD group, CHD with hypertension group, and during H7N9 or H1N1 infection. The number of infected individuals for each group was: day 0–7 group (H7N9:n=24; H1N1:n=10), day 8–14 group (H7N9:n=11; H1N1:n=7) and day 15 group (H7N9:n=11; H1N1:n=4). The horizontal lines represent the median value in each group. Detailed statistical information is shown inSupplementary Table 4. (b) Angiotensin II plasma levels at week 1 and week 2 in H7N9-infected patients hospitalized less than 28 days (n=11), hospitalized longer than 28 days (n=6) and deceased (n=5). The horizontal lines represent the mean value in each group. All experiments were in duplicate. Mann–WhineyUtest and Wilcoxon matched-pair test were used in the statistics. *P<0.05, **P<0.01, ***P<0.001. 1 , Table 1 ). We also collected plasma from 21 swine-origin influenza (H1N1) virus-infected patients in Beijing from December 2012 to February 2013 ( Supplementary Table 1 ). The presence of H7N9 and H1N1 influenza viruses was confirmed by PCR. Plasma from six healthy volunteers from the China CDC who were considered to be at high risk for H7N9 infection and plasma from 46 coronary heart disease (CHD) patients in Beijing were collected from April 2013 to June 2013. The characteristics of the study subjects are shown in Supplementary Tables 2–4 . To stratify the distinct time points during the illness, plasma was obtained within the first 7 days of disease onset (H7N9: n =24; H1N1: n =10), between 8 and 14 days following disease onset (H7N9: n =11; H1N1: n =7), and during the recovery phase from 15 days after disease onset (H7N9: n =11; H1N1: n =4) ( Fig. 1a ). Intriguingly, at all stages, angiotensin II plasma levels were markedly higher in H7N9-infected patients than in H1N1-infected patients, all CHD patients, and CHD patients with a diagnosis of hypertension ( Fig. 1a , Table 1 , Supplementary Tables 1–4 ). Angiotensin II levels in plasma from H1N1-infected patients obtained during the first week of disease were moderately higher than in those obtained from healthy individuals, whereas angiotensin II levels in plasma obtained during other time periods from H1N1-infected patients and CHD patients were not significantly different from those of high-risk healthy individuals ( Fig. 1a , Supplementary Table 4 ). Notably, angiotensin II levels decreased in H7N9-infected patient plasma harvested 15 days after disease onset, suggesting that angiotensin II levels may be related to disease severity in the early stage of avian influenza H7N9 infection ( Fig. 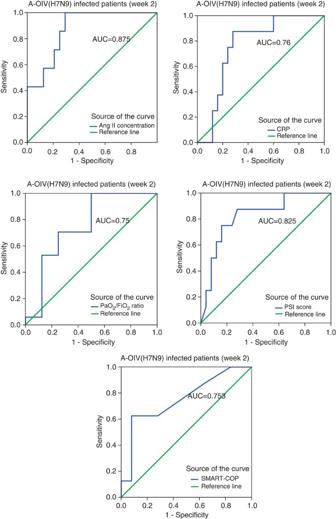Figure 4: Receiver operating characteristic (ROC) curve of plasma angiotensin II levels and other biomarkers during the second week of H7N9 infection. ROC curve of the plasma angiotensin II levels, C-reactive protein (CRP), PaO2/FiO2ratios, pneumonia severity index (PSI) scores and SMART-COP scores in the second week of avian-origin H7N9 Influenza A virus (A-OIV H7N9) infection are shown. Detailed information on the area under the ROC curve (AUC), the cut-off values, sensitivity, specificity, the positive predictive value (PPV), the negative predictive value (NPV), the positive likelihood ratio (PLR), the negative likelihood ratio (NLR) and Youden’s index are shown inSupplementary Tables 6–11. 1a , Supplementary Table 4 ). Table 1 Characteristics of the 35 patients with H7N9 virus infection. Full size table Figure 1: Angiotensin II levels are increased in plasmas of H7N9-infected patients. Among the study participants, 46 patients were infected with avian-origin H7N9 Influenza A virus (A-OIV H7N9) and 21 were infected with swine-origin H1N1 influenza A virus (S-OIV H1N1). In addition, six healthy volunteers, 46 CHD patients and 35 CHD patients with hypertension were recruited as controls. ( a ) Angiotensin II levels in plasma of healthy controls, CHD group, CHD with hypertension group, and during H7N9 or H1N1 infection. The number of infected individuals for each group was: day 0–7 group (H7N9: n =24; H1N1: n =10), day 8–14 group (H7N9: n =11; H1N1: n =7) and day 15 group (H7N9: n =11; H1N1: n =4). The horizontal lines represent the median value in each group. Detailed statistical information is shown in Supplementary Table 4 . ( b ) Angiotensin II plasma levels at week 1 and week 2 in H7N9-infected patients hospitalized less than 28 days ( n =11), hospitalized longer than 28 days ( n =6) and deceased ( n =5). The horizontal lines represent the mean value in each group. All experiments were in duplicate. Mann–Whiney U test and Wilcoxon matched-pair test were used in the statistics. * P <0.05, ** P <0.01, *** P <0.001. Full size image To investigate whether changes in angiotensin II levels among H7N9-infected patients are associated with disease progression and/or outcome, we analysed angiotensin II levels in 22 H7N9-infected patients for whom serially collected of plasma samples from both the first and second week of illness were available ( Fig. 1b ). These 22 H7N9-infected patients were divided into three groups according to disease outcome: patients who were discharged from the hospital within 28 days, patients who were discharged from the hospital after more than 28 days and patients who died ( Fig. 1b ). Interestingly, in the group of patients discharged from the hospital within 28 days, plasma angiotensin II levels significantly decreased during the second week of illness compared with the first week. However, in the group of patients hospitalized for a longer period or who died, plasma angiotensin II levels remained high during the second week of illness ( Fig. 1b ). Therefore, plasma angiotensin II levels in H7N9-infected patients may stratify disease severity and may be predictive of disease outcome. Angiotensin II levels are correlated with viral load We next analysed the potential correlation between patient plasma angiotensin II levels and viral load, APACHE II score and mortality using samples from a total of 35 H7N9-infected patients. These samples included the above mentioned 22 H7N9-infected patients with both week 1 and week 2 plasma samples plus two patients with week 1 samples only and 11 patients with week 2 plasma samples only. In parallel, we used viral cycle threshold (Ct) values from H1N1-infected patients (10 patient samples from week 1 and 7 patient samples from week 2) to calculate the correlation. To establish viral load, we collected pharyngeal samples on the same day as plasma collection from 21 H7N9 patients during the first week of illness and 30 H7N9 patients during the second week of illness. Viral loads were determined using Ct values for the H7N9-specific haemagglutinin gene by quantitative real-time reverse transcription-PCR as previously described [21] , [22] . We excluded samples with Ct values that indicated negative viral load. Pearson correlation analysis showed that plasma angiotensin II levels were indeed negatively correlated with H7N9 virus Ct values (and thus, positively correlated with viral load) during week 1, but not week 2 of illness ( Supplementary Table 5 ). Our data suggested that elevations of angiotensin II levels in the plasmas of H7N9-infected patients harvested during week 1 of disease onset were induced by avian influenza H7N9 virus. Interestingly, we also discovered a high linear correlation between H1N1 viral Ct value and angiotensin II levels in the plasma of patients infected with H1N1 collected at week 1 but not week 2 of disease onset ( Supplementary Table 5 ). Although the angiotensin II levels in plasmas from H1N1-infected patients were significantly lower than those in plasmas of H7N9-infected patients, the elevations of angiotensin II levels in plasmas harvested at the first week of disease onset was induced by swine-origin influenza virus H1N1 ( Supplementary Table 5 ). Angiotensin II levels are associated with disease severity APACHE II scores were determined to evaluate disease severity on the first day in the intensive care unit [19] , [20] . Plasma angiotensin II levels in H7N9 patients during the second week of illness demonstrated a high and significantly positive linear correlation with APACHE II scores, whereas angiotensin II levels during the first week of illness showed a weaker, albeit significant, positive linear correlation with disease severity ( Fig. 2 ). Again, plasma angiotensin II levels of H1N1-infected patients were positively correlated with patient APACHE II scores; however, the Spearman rank coefficient correlation did not pass hypothesis testing ( Supplementary Fig. 2 ). 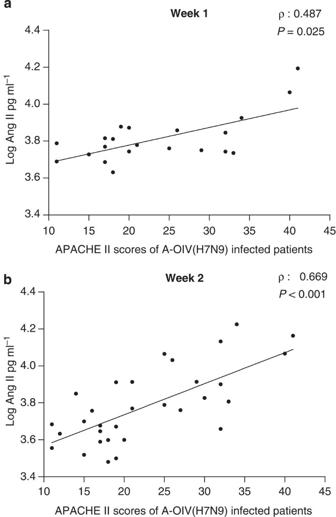Our results suggest a potential therapeutic strategy that would involve decreasing angiotensin II plasma levels during H7N9 infections. Figure 2: APACHE II scores are highly positively correlated with plasma angiotensin II levels in H7N9-infected patients. APACHE II scores from 21 and 32 avian-origin H7N9 Influenza A virus (A-OIV H7N9)-infected patients were available for the first and second week’s correlation analysis, respectively. Spearman rank correlation analysis (ρ) andPvalue are provided in each graph. Figure 2: APACHE II scores are highly positively correlated with plasma angiotensin II levels in H7N9-infected patients. APACHE II scores from 21 and 32 avian-origin H7N9 Influenza A virus (A-OIV H7N9)-infected patients were available for the first and second week’s correlation analysis, respectively. Spearman rank correlation analysis (ρ) and P value are provided in each graph. Full size image Angiotensin II levels at week 2 can predict fatal outcomes We further analysed whether angiotensin II levels were linked to fatal outcomes. Indeed, plasma angiotensin II levels during the second week of H7N9 illness were statistically significantly higher in the group of patients who died compared with the group who were discharged from the hospital within 28 days ( Fig. 3 ). Most swine-origin influenza A (H1N1) virus infections were not fatal. 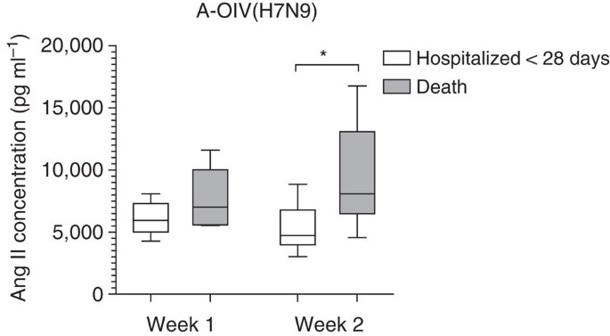Among the 21 H1N1-infected patients we studied, one patient died and 19 patients were released from the hospital within 28 days. Figure 3: Fatal outcome is linked to high plasma levels of angiotensin II in H7N9-infected patients. Angiotensin II concentrations in plasma from the first and second week of illness caused by avian-origin H7N9 Influenza A virus (A-OIV H7N9) in different outcome groups. The number of patients and the time-period in which they died are as follows. Patients with plasma harvested during the first week of illness: patients hospitalized less than 28 days (n=12), death (n=5). Patients with plasma harvested during the second week of illness: patients hospitalized less than 28 days (n=16), death (n=8). The horizontal lines represent the median value in each group. Mann–WhineyUtest was used in the statistics. *P<0.05. Figure 3: Fatal outcome is linked to high plasma levels of angiotensin II in H7N9-infected patients. Angiotensin II concentrations in plasma from the first and second week of illness caused by avian-origin H7N9 Influenza A virus (A-OIV H7N9) in different outcome groups. The number of patients and the time-period in which they died are as follows. Patients with plasma harvested during the first week of illness: patients hospitalized less than 28 days ( n =12), death ( n =5). Patients with plasma harvested during the second week of illness: patients hospitalized less than 28 days ( n =16), death ( n =8). The horizontal lines represent the median value in each group. Mann–Whiney U test was used in the statistics. * P <0.05. Full size image We performed biostatistical analyses to confirm angiotensin II as a biomarker of fatal outcome. We first used SPSS software to calculate its predictive value of fatal outcome ( Supplementary Table 6 ). In addition to angiotensin II, we also included a biomarker for infectious disease C-reactive protein, and clinical parameters of pneumonia severity index score and SMART-COP in the analysis [23] , [24] . The area under the curve of plasma angiotensin II levels during the second week of illness among H7N9-infected patients was 0.875, and the predictive values of C-reactive protein, pneumonia severity index score and SMART-COP were all less significant than angiotensin II ( Fig. 4 , Supplementary Table 6 ). Our data suggested that angiotensin II level at the week 2 of disease onset could predict the fatal outcome. We also used MedCalc software and the results were the same ( Supplementary Table 7 ). The sensitivity and specificity of this analysis were 87.5% and 68%, respectively ( Supplementary Table 7 ). In addition, the positive predictive value, negative predictive value, positive likelihood ratio and negative likelihood ratio within 95% confidence intervals were determined ( Supplementary Table 7 ). Figure 4: Receiver operating characteristic (ROC) curve of plasma angiotensin II levels and other biomarkers during the second week of H7N9 infection. ROC curve of the plasma angiotensin II levels, C-reactive protein (CRP), PaO 2 /FiO 2 ratios, pneumonia severity index (PSI) scores and SMART-COP scores in the second week of avian-origin H7N9 Influenza A virus (A-OIV H7N9) infection are shown. Detailed information on the area under the ROC curve (AUC), the cut-off values, sensitivity, specificity, the positive predictive value (PPV), the negative predictive value (NPV), the positive likelihood ratio (PLR), the negative likelihood ratio (NLR) and Youden’s index are shown in Supplementary Tables 6–11 . Full size image Using logistic regression analysis, we further analysed the independent predictor for fatal outcome among patients with H7N9 infections. Angiotensin II levels in plasma harvested during the second week of illness were determined to be an independent predictor among the clinical parameters of H7N9-infected patients including hypertension ( Table 2 ). Taken together, these results suggest that plasma angiotensin II levels, especially during the second week of illness, are an indicator of disease severity among H7N9-infected patients and are positively associated with mortality. Table 2 Logistic regression analysis of independence outcome predictor for plasma angiotensin II level independency in H7N9-infected patients during the second week of illness onset. Full size table Angiotensin II is an octapeptide that is a potent vasopressor and a powerful stimulus for the production and release of aldosterone from the adrenal cortex [25] , [26] , [27] , [28] , [29] . Angiotensin II is a major substrate of the RAS [29] , [30] , [31] . Previous studies have shown that RAS has important roles in cardiovascular disease, neurodegenerative disorders, and importantly, acute lung injury [16] , [32] , [33] , [34] , [35] , [36] , [37] , [38] , [39] . In our study, we reveal for the first time that angiotensin II levels in human blood are associated with H7N9-induced disease severity and may potentially predict patient mortality. However, the limitation of this study is its retrospective nature, and further studies of additional potential biomarkers in patient plasma are needed in the future. For historical reasons, there is currently no clinical biomarker to predict fatal outcome for lethal virus infection. In addition to the lack of a sufficiently sized cohort for standard statistical analysis, fatal outcomes usually result from multiorgan failure and are therefore difficult to associate with changes in a single protein in human plasma. Angiotensin II in the RAS has functions in multiple organs; it is indeed a likely biomarker that can be used to predict fatal outcome in lethal diseases. Together with our accompanying paper describing treatment options [18] , these results raise the intriguing possibility that therapies targeting RAS may represent viable strategies for treating this deadly disease. In addition to recombinant human angiotensin-converting enzyme 2 (in clinical trial), angiotensin II lowering drugs, including ACE inhibitors and angiotensin II receptor blockers, are clinically available [40] , [41] . Future studies are necessary to determine the therapeutic effects of the proposed RAS targeting drugs in lethal virus infections. Clinical specimens H7N9-infected patients were recruited at the First Affiliated Hospital, College of Medicine, Zhejiang University ( n =40), Jiangsu province ( n =6) and Shanghai city ( n =1). H1N1-infected patients were recruited from December 2012 to February 2013 at Beijing Chao-yang Hospital, Capital Medical University ( n =21). Six healthy volunteers who were considered at high risk for H7N9 infection by the Chinese Center for Disease Control and Prevention (China CDC) and 46 CHD patients, including 35 CHD patients with a diagnosis of hypertension, from Peking Union Medical College Hospital (PUMCH) during the same period were recruited as controls. Clinical information was collected by attending physicians on the same day as plasma sampling. Basic clinical information and treatments are shown in Table 1 , Supplementary Tables 1–4 . Blood samples were collected using EDTA-anticoagulant tubes and centrifuged to obtain the plasma. H7N9-infected patient plasma was collected at least twice while in the hospital, including where possible one sample during the first week and one sample during the second week of illness onset after admission to the hospital. Patient sputum was collected on the same day. We used TaqMan real-time reverse transcription-PCR under standard thermal cycling conditions to detect M, H7, and N9 genes specific to the H7N9 influenza virus and H1 and N1 genes specific to the H1N1 influenza virus [1] , [42] , [43] . All specimens were stored at −80 °C until analysis. Informed written consents were obtained from all participants before enrolment in the study. This study conformed to the ethical guidelines of the 1975 Declaration of Helsinki and was approved by the Institutional Review Board of the First Affiliated Hospital of Zhejiang University, Beijing Chao-yang Hospital, China CDC and PUMCH. Measurement of angiotensin II in patient plasma The plasma concentration of angiotensin II was measured by ELISA according to the manufacturer’s instructions (RapidBio Lab, USA). All experiments were performed in a biosafety level 2 laboratory and in duplicates. Statistical analysis The Mann–Whitney U test or χ 2 -test was used to determine differences between two groups. Wilcoxon matched-pair tests were employed to assess differences between the first and the second week of disease onset among the same patients. The Pearson correlation coefficient and Spearman rank correlation coefficient were used for linear correlation analysis. We calculated receiver operating characteristic curves for predictive analysis. Logistic regression was used for independent predictor analysis. Mann–Whitney U test, χ 2 -test, Wilcoxon matched-pair test, Pearson correlation coefficient analysis, Spearman rank correlation coefficient analysis and Logistic regression analysis were performed with SPSS 16.0 for Windows (SPSS, Inc.). Receiver operating characteristic curves calculation was performed with SPSS 16.0 for Windows and MedCalc Software. A P -value<0.05 was considered statistically significant. How to cite this article: Huang, F. et al. Angiotensin II plasma levels are linked to disease severity and predict fatal outcomes in H7N9-infected patients. Nat. Commun. 5:3595 doi: 10.1038/ncomms4595 (2014).